Strain and curvature induced evolution of electronic band structures in twisted graphene bilayer It is well established that strain and geometry could affect the band structure of graphene monolayer dramatically. Here we study the evolution of local electronic properties of a twisted graphene bilayer induced by a strain and a high curvature, which are found to strongly affect the local band structures of the twisted graphene bilayer. The energy difference of the two low-energy van Hove singularities decreases with increasing lattice deformation and the states condensed into well-defined pseudo-Landau levels, which mimic the quantization of massive chiral fermions in a magnetic field of about 100 T, along a graphene wrinkle. The joint effect of strain and out-of-plane distortion in the graphene wrinkle also results in a valley polarization with a significant gap. These results suggest that strained graphene bilayer could be an ideal platform to realize the high-temperature zero-field quantum valley Hall effect. Graphene, a material made of a two-dimensional honeycomb carbon lattice, is acting as a bridge between quantum field theory and condensed matter physics owing to its gapless, massless and chiral Dirac spectrum [1] , [2] . Graphene’s two-dimensional nature makes it amenable to external mechanical deformation. It is now well established that lattice deformations of graphene lead to the appearance of a pseudomagnetic gauge field acting on the charge carriers [2] , [3] , [4] , [5] , [6] , [7] , [8] , [9] , [10] . The pseudomagnetic field becomes an experimental reality after the observation of Landau levels (LLs) in a strained graphene monolayer [11] , [12] , [13] , [14] and in strained artificial graphene [15] . The energies of these LLs follow the progression of LLs of massless Dirac Fermions, which suggest a possible route to realize zero-field quantum Hall effects in the strained graphene [11] , [12] , [13] , [14] , [15] . Compared with single-layer graphene, graphene bilayers, including AA stacked, AB stacked (Bernal) and twisted graphene bilayer, display even more complex electronic band structures and intriguing properties because of the interplay of quasiparticles between the Dirac cones on each layer [16] , [17] , [18] , [19] , [20] , [21] , [22] , [23] , [24] , [25] , [26] , [27] , [28] . Recently, several groups addressed the physics of the strained graphene bilayer (either AA- or AB-stacked graphene bilayer) theoretically and obtained many interesting results [29] , [30] , [31] , [32] , [33] , [34] . Despite many suggestive findings and potential applications, there have unfortunately been no experimental studies of the effect of strain on the electronic band structures of the graphene bilayer. In this article, we report the local electronic properties of a corrugated twisted graphene bilayer with a twist angle θ~5.1° studied by scanning tunnelling microscopy and spectroscopy (STM and STS). In the flat region of the sample, we observe two low-energy van Hove singularities (VHSs), which originate from two saddle points flanking the Dirac points of the band structure [20] , [22] , [23] , [26] , [27] , and superlattice Dirac points generated by the graphene-on-graphene moiré. Around a wrinkle of the twisted graphene bilayer, the moderate lattice deformations and the possible enhanced interlayer coupling lead to the decrease of the energy difference of the two VHSs. Remarkably, we observe apparent zero-field LL-like quantizations, which mimic the quantizations of massive chiral Fermions of Bernal graphene bilayer in a perpendicular magnetic field of about 100 T, along the strained wrinkle. We also show that the strain and curvature result in a valley polarization of the twisted graphene bilayer, that is, the eightfold degenerate LL at the charge neutrality point is splitted into two fourfold degenerate quartets polarized on each layer with a significant gap. Our experimental result suggests that the strained twisted graphene bilayer could be an ideal platform to realize zero-field quantum valley Hall effect [35] , [36] . Strained twisted graphene bilayer around a Rh step edge The twisted graphene bilayer was grown on a 25-μm-thin Rh foil via a traditional ambient pressure chemical vapour deposition method [26] , and only the sample mainly covered with two graphene layers was further studied by STM and STS. Owing to the thermal expansion mismatch between graphene and the substrate, defect-like wrinkles and ripples tend to evolve along the boundaries of crystalline terraces for a strain relief [11] , [14] , [37] , [38] . Briefly, the sample was synthesized at 1,000 °C and after growth when the sample is cooled down the graphene expands while the Rh foil contracts. As a consequence, strain builds up in the sample and the graphene wrinkles are induced at the step edges of Rh foil where the graphene is possibly weakly coupled to the Rh. 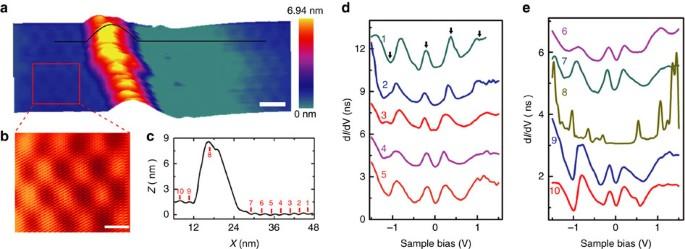Figure 1: STM images and STS of twisted graphene bilayer. (a) Large-area STM image of a twisted graphene bilayer with a wrinkle along a step of the Rh foil (Vsample=−600 mV andI=0.24 nA). Moiré pattern with identical period appears on both the right and left terraces flanking the wrinkle. The white scale bar is 5 nm. (b) Atomic-resolution image of the twisted graphene bilayer in the red frame of panel (a). It shows a moiré pattern with the period of 2.76 nm (Vsample=−351 mV andI=0.14 nA). The white scale bar is 2 nm. The twisted angle of the graphene bilayer is estimated as about 5.1o. (c) A line profile along the black curve in panel (a). The average height and width (peak width at half-height) of the wrinkle are about 7.9 and 8.2 nm, respectively. The small periodic protuberances with a period of about 2.76 nm on the two terraces are attributed to the moiré pattern. STS measurements at different positions along the line profile show quite different characteristics, as shown in (d) and (e). The spectra have been vertically offset for clarity. Curves 1, 2, 3, 4, 5, 6, 7, 9 and 10 are measured on the flat twisted graphene bilayer. The two peaks flanking the Dirac point, as pointed out by the arrows, are attributed to the two VHSs. The two dips pointed out by the arrows are the positions of the superlattice Dirac points generated by the graphene-on-graphene moiré. The sharp peaks in curve 8 are attributed to the Landau quantizations of the strained graphene bilayer in a large pseudomagnetic field. Figure 1a shows a typical STM image of a graphene wrinkle at the boundary of two flat terraces of the Rh surface. Moiré patterns with identical period of ~2.76 nm are observed on both the right and left terraces flanking the wrinkle, as shown in Fig. 1b . For monolayer graphene on a Rh(111) surface, the lattice mismatch between graphene (0.246 nm) and Rh(111) (0.269 nm) leads to hexagonal moiré superstructures with the expected periodicity approximately about 2.9 nm resulted from a 12C/11Rh coincidence lattice [39] , [40] , [41] ( Supplementary Fig. S1 , the characteristic of the moiré superstructures is distinct from that shown in Fig. 1 ). The 2.76 nm periodic protuberance, as shown in Fig. 1 , is attributed to the moiré pattern arising from a stacking misorientation between the top graphene layer and the underlayer graphene. The twisted angle θ, estimated as 5.1°, is related to the period of the moiré pattern by D = a /[2sin(θ/2)] with a ~0.246 nm. The line profile, as shown in Fig. 1c , indicates that the one-dimensional wrinkle is a strained structure of the twisted graphene bilayer with a high curvature and out-of-plane distortions at the apex (see Supplementary Fig. S2 for a STM topography of the wrinkle). The average height and width (peak width at half-height) of the wrinkle are about 7.9 and 8.2 nm, respectively. For a corrugated twisted graphene bilayer with a small curvature, we can observe moiré superstructures along wrinkles and ripples [37] , [38] ( Supplementary Fig. S3 ). However, it is difficult to obtain atomic-resolution image of the wrinkle shown in Fig. 1 because of its large curvature. The wrinkle could still be twisted graphene bilayer with a finite interlayer coupling and, of course, the large bending of the wrinkle also can result in a local slide of two graphene sheets relative to each other, then the two graphene sheets may become decoupled at the very top of the wrinkle. Figure 1: STM images and STS of twisted graphene bilayer. ( a ) Large-area STM image of a twisted graphene bilayer with a wrinkle along a step of the Rh foil ( V sample =−600 mV and I =0.24 nA). Moiré pattern with identical period appears on both the right and left terraces flanking the wrinkle. The white scale bar is 5 nm. ( b ) Atomic-resolution image of the twisted graphene bilayer in the red frame of panel ( a ). It shows a moiré pattern with the period of 2.76 nm ( V sample =−351 mV and I =0.14 nA). The white scale bar is 2 nm. The twisted angle of the graphene bilayer is estimated as about 5.1 o . ( c ) A line profile along the black curve in panel ( a ). The average height and width (peak width at half-height) of the wrinkle are about 7.9 and 8.2 nm, respectively. The small periodic protuberances with a period of about 2.76 nm on the two terraces are attributed to the moiré pattern. STS measurements at different positions along the line profile show quite different characteristics, as shown in ( d ) and ( e ). The spectra have been vertically offset for clarity. Curves 1, 2, 3, 4, 5, 6, 7, 9 and 10 are measured on the flat twisted graphene bilayer. The two peaks flanking the Dirac point, as pointed out by the arrows, are attributed to the two VHSs. The two dips pointed out by the arrows are the positions of the superlattice Dirac points generated by the graphene-on-graphene moiré. The sharp peaks in curve 8 are attributed to the Landau quantizations of the strained graphene bilayer in a large pseudomagnetic field. Full size image VHSs and superlattice Dirac points Figure 1d show ten d I /d V−V curves recorded at different positions along the line profile in Fig. 1c . Curves 1–7, 9 and 10 are measured at the flat twisted graphene bilayer on the Rh terraces. Curve 8, which shows distinct characteristics comparing with that of the curves 1–7, 9 and 10, is measured at the strained wrinkle. The tunnelling spectrum gives direct access to the local density of states (LDOSs) of the surface at the position of the STM tip. The experimental result in Fig. 1d indicates that the strain affects the electronic band structures of the twisted graphene bilayer remarkably. For a twisted graphene bilayer, the Dirac points of the two layers no longer coincide and the zero-energy states occur at k =−Δ K /2 in layer 1 and k =Δ K /2 in layer 2 (here | ΔK |=Δ K =2 K sin(θ/2) is the shift between the corresponding Dirac points of the twisted graphene bilayer, and K =4π/3 a with a ~0.246 nm the lattice constant of the hexagonal lattice). When there is a finite interlayer hopping t θ , two saddle points (two VHSs) at Δ E vhs = ħ ν F Δ K −2 t θ are unavoidable along the intersection of the two Dirac cones: K and K θ (refs 22 , 23 , 26 , 42 , 43 ) ( Supplementary Fig. S4 and Supplementary Note 1 ). The two pronounced peaks flanking zero-bias in the tunnelling spectra of the curves 1–7, 9 and 10, as shown in Fig. 1 , are attributed to the two VHSs of the LDOSs. For a twisted graphene bilayer with a vanishingly small interlayer coupling, one can only observe the moiré pattern but not the VHSs in the STM studies [22] . In our experiment, the energy difference of the two VHSs Δ E vhs deduced from the tunnelling spectra is almost a constant at a fixed position. However, the energy difference of the two peaks decreases when the experimental position approaches the strained wrinkle (similar experimental result was also observed in the left terraces of the wrinkle). For the curve 1, the energy difference of the two VHSs is Δ E vhs ~0.59 eV. For the curve 7, the value of Δ E vhs decreases to 0.38 eV, as shown in Supplementary Fig. S5 . We will demonstrate subsequently that the decrease of Δ E vhs originates from the strain-induced lattice deformations. Besides the two VHSs, the curves 1−7, 9 and 10 show two dips in the LDOSs (marked by arrows), symmetrically placed at about ±(1.05±0.05) eV around the graphene Dirac point, irrespective of the experimental positions, but generally of asymmetric strength. This reminds us the characteristic of superlattice Dirac points at E SD ~± h ν F | G |/2 in both graphene monolayer and twisted graphene bilayer induced by a weak periodic potential (experimentally, the periodic potential can be generated by the moiré pattern between the top layer graphene and the substrate (or the under layer graphene); here G is the reciprocal superlattice vectors of the moiré pattern) [44] , [45] , [46] , [47] , [48] , [49] . The graphene-on-graphene moiré pattern can provide a weak periodic potential, which leads to the emergence of the superlattice Dirac points [49] , [50] . Considering the period of the moiré pattern of ~2.76 nm and ν F ~1.1 × 10 6 m s −1 , we obtain E SD ~±0.95 eV, which is slightly smaller than our experimental value (see Supplementary Fig. S6 and Supplementary Note 2 for the theoretical model of the emergence of superlattice Dirac points in the twisted graphene bilayer). This slight discrepancy may arise from the fact that the value of velocity far from the charge neutrality point of graphene is larger than 1.1 × 10 6 m s −1 . It could reach (1.5±0.2) × 10 6 m s −1 (ref. 51 ). LL quantizations and valley polarization Now we turn to understand the distinct spectrum obtained at the strained wrinkle, shown as the curve 8 in Fig. 1 . The sharp peaks of the tunnelling spectrum are attributed to the LLs of the strained graphene wrinkle. The large strain stress and out-of-plane distortions of the graphene wrinkle can result in a large pseudomagnetic field on its electronic structures [52] , [53] , [54] , [55] . Our analysis is summarized in Fig. 2 . It is shown that these LLs follow the progression of LLs of the massive chiral fermions E N =± { ħω c [ N ( N -1)] 1/2 + E g /2}, N =0,1,2,…. (Here ω c = e B S / m * is the cyclotron frequency, B S is the pseudomagnetic field, m * =0.03 m e with m e the mass of electron and E g ~0.32 eV is the band gap) [16] , [18] . The energy of the pseudo-LLs as a function of the orbital and valley index ( N , ξ ) are plotted in Fig. 2d . It shows that our experimental data match the equation perfectly. The pseudomagnetic field of the strained wrinkle estimated according to the spectrum is about 100 T. The wrinkle is one of the simplest model to study the strain-induced pseudo-magnetic flux of a corrugated graphene sheet [7] . The flux of the wrinkle can be estimated by Φ =( βh 2 / la ) Φ 0 (here h is the height, l is the width of the wrinkle, 2< β <3, a is on the order of the C–C bond length and Φ 0 is the flux quantum) [7] , [11] , [12] . It is unexpected that the strain-induced LL-like quantizations of the twisted graphene bilayer are identical to the Landau quantizations of the massive chiral Fermions in Bernal stacking graphene bilayer in an external magnetic field [16] . This result suggests that the corrugated structure modifies structure of the twisted graphene bilayer along the wrinkle efficiently, which as a consequence results in the massive chiral fermions (where the electronic energy dispersion is hyperbolic in momentum) of the strained wrinkle. We will demonstrate subsequently that the strain and the large curvature could lead to a hyperbolic band structure of the graphene wrinkle. 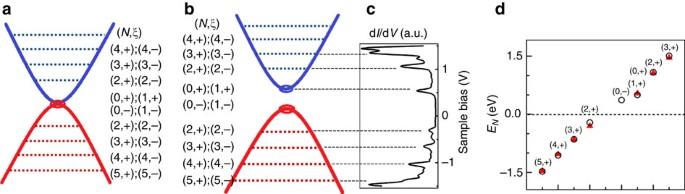Figure 2: Landau quantizations of the massive chiral fermions. The formation of LLs of massive chiral fermions in the quantum Hall regime (a) without and (b) with a band gap. LLs are indexed by the orbital and valley index, (N,ξ) (ξ=+1 for valleyK,ξ=−1 for valleyK′). When there is a gap, the eightfold degenerate level at the charge neutrality point becomes layer-polarized quartets. The LL(0,+);(1,+)projected on the top layer and the LL(0,−);(1,−)on the underlayer graphene. (c) The tunnelling spectrum at the strained wrinkle. The sharp peaks are attributed to the LLs. The energies of these LLs follow the progression of LLs of the massive chiral Fermions with a band gap. The pseudomagnetic field is estimated as 100 T and the gap of the valley polarization is about 0.32 eV. (d) The pseudo-LLs (the solid triangles) of the experimental data in (c) as a function of the orbital and valley index (N,ξ). The open circles show the progression of LLs of massive chiral FermionsEN=±{ħωc[N(N-1)]1/2+Eg/2}, N=0,1,2,…… Figure 2: Landau quantizations of the massive chiral fermions. The formation of LLs of massive chiral fermions in the quantum Hall regime ( a ) without and ( b ) with a band gap. LLs are indexed by the orbital and valley index, ( N , ξ ) ( ξ =+1 for valley K , ξ =−1 for valley K′ ). When there is a gap, the eightfold degenerate level at the charge neutrality point becomes layer-polarized quartets. The LL (0,+);(1,+) projected on the top layer and the LL (0,−);(1,−) on the underlayer graphene. ( c ) The tunnelling spectrum at the strained wrinkle. The sharp peaks are attributed to the LLs. The energies of these LLs follow the progression of LLs of the massive chiral Fermions with a band gap. The pseudomagnetic field is estimated as 100 T and the gap of the valley polarization is about 0.32 eV. ( d ) The pseudo-LLs (the solid triangles) of the experimental data in ( c ) as a function of the orbital and valley index ( N , ξ ). The open circles show the progression of LLs of massive chiral Fermions E N =± { ħω c [ N ( N -1)] 1/2 +E g /2} , N= 0,1,2,…… Full size image The size of the LL wavefunction, that is, the magnetic length l B =[ ħ /( e B )] 1/2 , generated by the pseudomagnetic field (~100 T) is about 2.6 nm, which is much smaller than the size of the graphene wrinkle. The difference between on-site potential (the staggered potential) of the A and B atoms in the two graphene sheets becomes important along the graphene wrinkle [25] . Therefore, it is expected that the eightfold degenerate LL at the charge neutrality point could be locally lifted by the pseudomagnetic field. In our experiment, the eightfold degenerate LL at the charge neutrality point is splitted into two fourfold degenerate quartets polarized on each layer with a gap E g ~0.32 eV. Importantly, the N =0 and N =1 states LL (0,+);(1,+) in the K valley (labelled as ξ =+1) are localized predominantly on the B sites of the top layer, whereas the N =0 and N =1 states LL (0,−);(1,−) in the K′ valley (labelled as ξ =−1) are localized predominantly on the A sites of the underlayer graphene [25] . Therefore, it is not surprising that only LL (0,+);(1,+) in the K valley, which is polarized on the top layer, could be observed by the STS measurement, as shown in Fig. 2 . The energy interval with zero tunnelling DOS around the Fermi level of the spectrum is therefore the sum of the energy gap and the energy difference between the LL (0,-);(1,-) and LL (2,+);(2,-) . As discussed in the preceding chapter, the large bending of the wrinkle may decouple the two graphene sheets at the very top of the wrinkle. Then we can observe single-layer behaviours of the wrinkle. For the case that the joint effect of the strain and curvature is not strong enough to generate a band gap, then the degeneracy of the LL (0,+);(1,+) and LL (0,−);(1,−) states is not lifted and it is expected to observe Landau-level quantizations of massless Dirac fermions in the wrinkle, as observed in strained graphene monolayer in refs 11 , 12 , 13 , 14 . For the case that the corrugated structure has a large strain and curvature, then the joint effect could open a gap and generate a hyperbolic energy dispersion in graphene monolayer [4] , and simultaneously the non-uniform strain can induce the Landau-levels characteristic of massive chiral fermions. However, in this case, it is expected to observe both the LL (0,+);(1,+) and LL (0,−);(1,−) states in the STS spectrum. Obviously, the results of the above two cases are in stark contradiction to that of our experiment. Therefore, it is reasonble to assume that the studied wrinkle is a twisted graphene bilayer with a finite interlayer coupling and consequently we observed valley polarization on each layer. Very recently, it is predicted that the valley-polarized quantum Hall phases can be driven by Coulomb interaction in strained graphene [56] . The observed valley polarization (with the energy gap of ~0.32 eV) on each layer and large pseudomagnetic field suggest that the strained twisted graphene bilayer is an ideal platform to realize high-temperature zero-field quantum valley Hall effect. To further understand our experimental result, we calculated the effects of both the strain and curvature on the electronic band structures of the twisted graphene bilayer by tight-binding model with the Hamiltonian H=H 1 +H 2 + , where H 1 and H 2 are the Hamiltonians for each layer and is the interaction Hamiltonian between the two layers [20] , [42] , [57] . In the flat region around the wrinkle, the lattices of the twisted graphene bilayer are compressed several percentages in a prescribed direction and the out-of-plane distortion of the sample is very small. Therefore, we only consider the effect of a tensional strain on the electronic structure of the flat twisted graphene bilayer. 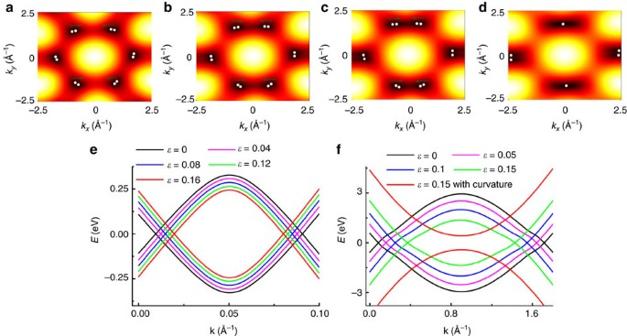Figure 3: Electronic band structures of twisted graphene bilayer. Density plots of the energy dispersion of twisted graphene bilayer for (a) {ε=0,θ=5.1o}, (b) {ε=0.1,θ=5.1o}, (c) {ε=0.15,θ=5.1o} and (d) {ε=0.15,θ=5.1o} with a curvature radius of ~1.41 nm at the top of the wrinkle. The white points are the four Dirac points:K,Kθ,K′andKθ′. In panel (e) we have a cut of the electronic band structures alongKandKθ, showing the decreasing of ΔEvhsas strain increases (in a small and moderate strain). In panel (f), we have a cut of the electronic band structures alongKandKθ′, showing the merging of the Dirac cones as the strain increases and the ultimate appearance of the gap induced by the joint effect of the strain and the curvature. Figure 3a–c shows the energy dispersions of the twisted graphene bilayer with different lattice deformations. With increasing lattice deformations and the variation of the nearest-neighbour hopping parameters, the Dirac points move away from the corners K and K′ , as shown in Fig. 3e . Figure 3: Electronic band structures of twisted graphene bilayer. Density plots of the energy dispersion of twisted graphene bilayer for ( a ) { ε =0, θ =5.1 o }, ( b ) { ε =0.1, θ =5.1 o }, ( c ) { ε =0.15, θ =5.1 o } and ( d ) { ε =0.15, θ =5.1 o } with a curvature radius of ~1.41 nm at the top of the wrinkle. The white points are the four Dirac points: K , K θ , K′ and K θ ′ . In panel ( e ) we have a cut of the electronic band structures along K and K θ , showing the decreasing of Δ E vhs as strain increases (in a small and moderate strain). In panel ( f ), we have a cut of the electronic band structures along K and K θ ′ , showing the merging of the Dirac cones as the strain increases and the ultimate appearance of the gap induced by the joint effect of the strain and the curvature. Full size image On the top of the wrinkle, the large bending causes rehybridization between π and σ orbitals of graphene and influences the Slater–Koster overlap integral [1] , [6] , [52] , [57] , [58] . Therefore, both the effect of the strain and the curvature should be considerated in the calculation (see Supplementary Note 3 for details). The large curvature at the top of the wrinkle could merge the Dirac points K and K′ into a single one ( Fig. 3d ). As a consequence, the LL-like quantizations in the graphene wrinkle should be identical to the Landau quantizations of the massive chiral Fermions in Bernal stacking graphene bilayer (as shown in Fig. 2 ). A band gap appears in the energy spectrum of the graphene wrinkle, as shown in Fig. 3f . This provides a physical mechanism to open a significant energy gap in the twisted graphene bilayer where an external electric field cannot open a gap in its spectrum [20] . We fit the section line of the wrinkle by a Gaussian curve to estimate its curvature, as shown in Fig. 4a . The joint effects of a considerable lattice deformation and the large curvature result in an almost hyperbolic electronic band of the wrinkle ( Fig. 3f ). 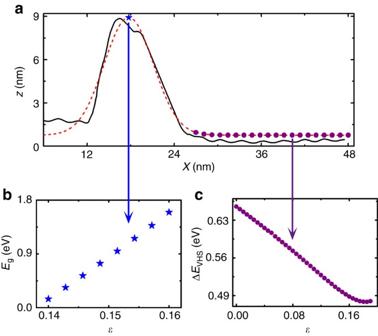Figure 4: Energy gap and ΔEvhsas a function of strain. In panel (a), the red dash line corresponds to a Gaussian fitting to the section line of the graphene wrinkle, as shown inFig. 1c. Panel (b) shows that the energy gap increases as the strain increases for a fixed curvature radius of ~1.41 nm at the top of the wrinkle. Panel (c) shows the value of ΔEvhsas a function of the strain in flat twisted graphene bilayer. Figure 4b shows the energy gap E g as a function of the strain for a fixed curvature radius of ~1.41 nm. The large curvature at the top of the wrinkle opens an energy gap in twisted graphene bilayer when the amount of strain ε reaches about 0.14. Figure 4c summarizes the value of Δ E vhs of the flat twisted graphene bilayer as a function of the tensional strain. In small and moderate deformations, the energy difference of the two VHSs Δ E vhs decreases as the strain increases, which agrees well with our experimental result. Figure 4: Energy gap and Δ E vhs as a function of strain. In panel ( a ), the red dash line corresponds to a Gaussian fitting to the section line of the graphene wrinkle, as shown in Fig. 1c . Panel ( b ) shows that the energy gap increases as the strain increases for a fixed curvature radius of ~1.41 nm at the top of the wrinkle. Panel ( c ) shows the value of Δ E vhs as a function of the strain in flat twisted graphene bilayer. Full size image The pseudo-Landau quantizations observed in our experiment may be induced by the local non-uniform strains as that the strained structure is quite rough along the wrinkle ( Supplementary Fig. S2 ). Usually, a constant pseudomagnetic field can be achieved when the honeycomb lattice are transversely displaced from their original positions in the following way ( u r , u φ )= qr 2 (sin3 φ ,cos3 φ ), where u r and u φ are the radial and azimuthal displacements, φ is the azimuthal angle, r is the distance from anbitrary origin and q is a parameter corresponding to the strength of the strain [8] , [11] , [12] , [13] , [14] . This uniform pseudomagnetic field is not easy to realize in the strained graphene [11] , [12] , [13] , [14] . Our experiment also confirms that the pseudomagnetic field is not uniform along the wrinkle ( Supplementary Fig. S7 ). However, the non-uniform strains can generate large local pseudomagnetic fields, which can be detected by the STS measurements along the wrinkle. Theoretically, it was predicted that the pseudo-Landau quantizations can be observed in corrugated graphene structure when the effective pseudomagnetic flux per wrinkle Φ ~( h 2 / la ) Φ 0 is larger than the flux quantum [5] , [6] . This condition is very difficult to satisfy for both the corrugated graphene monolayer and bilayer, as shown in Fig. 5 and the Methods section for detailed discussion. For the case that h 2 / la <1, the obtained STS spectra are almost identical to that of flat graphene monolayer ( Supplementary Fig. S8 ) and flat twisted graphene bilayer, respectively. For the corrugated structure that satisfies h 2 / la >1, the pseudo-LLs are observed. For the monolayer graphene wrinkle that satisfies h 2 / la >1, as shown in Fig. 5 , we only observed Landau-level quantizations of massless Dirac fermions (see Supplementary Fig. S9 and ref. 14 for more details). It indicates that the joint effect of the strain and curvature is not strong enough to generate a band gap in the monolayer graphene wrinkle. In the monolayer graphene wrinkle, h 2 / la ~3, whereas in the twisted bilayer wrinkle studied in this work, h 2 / la ~8. Therefore, our experimental result suggests that the effect of the curvature has a vital role for the emergence of the valley polarization in the twisted graphene bilayer. Further experiments by using substrate with predefined structures may be helpful to control the curvature of the corrugated graphene and induce the necessary strained wrinkles. 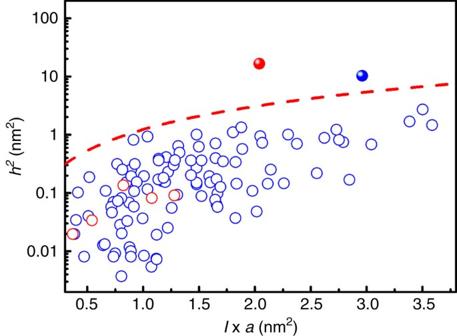Figure 5: Parameters of the graphene wrinkles studied in this work. The parameters,landh, of both the graphene monolayer wrinkles (blue circles) and graphene bilayer wrinkles (red circles) studied in our experiment. The filled circle represents the wrinkles showing LLs and the open circles are denoted by the wrinkles that do not show any evidence of the LL. The red dashed curve is plotted according toh2/la=1. Figure 5: Parameters of the graphene wrinkles studied in this work. The parameters, l and h , of both the graphene monolayer wrinkles (blue circles) and graphene bilayer wrinkles (red circles) studied in our experiment. The filled circle represents the wrinkles showing LLs and the open circles are denoted by the wrinkles that do not show any evidence of the LL. The red dashed curve is plotted according to h 2 /la =1. Full size image In summary, we studied the local electronic properties of the strained graphene bilayer with a twist angle of ~5.1°. Our experiment demonstrated that the energy difference of the two VHSs Δ E vhs decreases as the strain increases. Along the wrinkle of the twisted bilayer graphene, we observed apparent zero-field LL-like quantizations and the valley polarization with a large gap. The observed valley polarization on each layer, and large pseudomagnetic field of ~100 T suggest that the strained graphene bilayer is an ideal platform to realize high-temperature zero-field quantum valley Hall effect. Further effort should be made to generate large-scale strained graphene bilayer with a uniform pseudomagnetic field to carry out the transport measurements in this interesting system. Preparation of bilayer graphene on Rh foil The graphene bilayer was grown on a 25-μm-thin Rh foil via a traditional ambient pressure chemical vapour deposition method [26] . The process is similar to the systhesis of graphene on Pt and Cu foils, which were reported in previous papers [37] , [38] . Briefly, the Rh foil was first heated from room temperature to 1,000 °C for 45 min under an Ar flow of 850 s.c.c.m. Then the furnace was experienced a hydrogen gas flow of 50 s.c.c.m. for 40 min at 1,000 °C. Finally, CH 4 gas was introduced with a flow ratio of 5–10 s.c.c.m., and the growth time is varied from 3 to 15 min for controlling the thickness of graphene. The as-grown sample is cooled down to room temperature and can be transferred into the ultra-high vacuum condition for further characterizations. The thickness of the as-grown graphene was characterized by Raman spectra measurements [26] , and only the sample mainly covered with graphene bilayer was further studied by STM and STS. The Raman spectroscopy for the sample used here is shown in Supplementary Fig. S1 of ref. 26 . In previous papers, we studied carefully the structures and the formation mechanism of the wrinkles and ripples on metallic substrates [37] , [38] . In this paper, we focus on the local electronic properties of the wrinkles of the twisted graphene bilayer. STM and STS measurements The STM system was an ultra-high vacuum four-probe SPM from UNISOKU. All STM and STS measurements were performed at liquid-nitrogen temperature and the images were taken in a constant-current scanning mode. The STM tips were obtained by chemical etching from a wire of Pt (80%) Ir (20%) alloys. Lateral dimensions observed in the STM images were calibrated using a standard graphene lattice. The STS spectrum, that is, the dI/dV-V curve, was carried out with a standard lock-in technique using a 957 Hz a.c. modulation of the bias voltage. Tight-binding calculations All the calculations were based on tight-binding theories. The interlayer Hamiltonian of twisted graphene bilayer reads The strain and curvature can change the Slater–Koster overlap integral and modify the hopping parameters, which obey the following two formulas Based on the revised hopping parameters, as shown in Supplementary Note 3 , the Hamiltonian matrix in the four-component spinor representation is obtained. The band structure of the corrugated twisted bilayer graphene can be calculated through diagonalizing the 4 × 4 Hamiltonian matrix. The condition to satisfy h 2 / la ≥1 for corrugated graphene On the assumption that the wrinkles are generated in the presence of a longitudinal tensile strain , then, according to classical elasticity theory, the amplitude h and the period l can be obtained as [14] Here v is the Poisson ratio, t is the thickness of graphene and L is the length of a wrinkle. Then we can obtain The condition h 2 /la≥ 1 is satisfied when the length of the wrinkles L≥ 8 μm. Therefore, it is not very easy to observe the pseudo-LLs in graphene wrinkles. How to cite this article: Yan, W. et al. Strain and curvature induced evolution of electronic band structures in twisted graphene bilayer. Nat. Commun. 4:2159 doi: 10.1038/ncomms3159 (2013).